Adenosine is required for sustained inflammasome activation via the A2Areceptor and the HIF-1α pathway Inflammasome pathways are important in chronic diseases; however, it is not known how the signalling is sustained after initiation. Inflammasome activation is dependent on stimuli such as lipopolysaccharide (LPS) and ATP that provide two distinct signals resulting in rapid production of interleukin (IL)-1β, with the lack of response to repeat stimulation. Here we report that adenosine is a key regulator of inflammasome activity, increasing the duration of the inflammatory response via the A 2A receptor. Adenosine does not replace signals provided by stimuli such as LPS or ATP but sustains inflammasome activity via a cAMP/PKA/CREB/HIF-1α pathway. In the setting of the lack of IL-1β responses after previous exposure to LPS, adenosine can supersede this tolerogenic state and drive IL-1β production. These data reveal that inflammasome activity is sustained, after initial activation, by A 2A receptor-mediated signalling. The production of interleukin (IL)-1β is a central step in a wide range of acute and chronic inflammatory and fibrotic responses. The identification of the molecules that form the inflammasome has been a significant advance in our understanding of the required cytosolic machinery and upstream signals for IL-1β production [1] . Two distinct pathways are known to be required for initial inflammasome activation and IL-1β production. The signal 1 pathway is typically considered to be activated via Toll-like receptors resulting in NF-kβ-mediated upregulation of the Pro-ILβ gene, as well as genes for inflammasome components [2] . A second pathway (signal 2) is required for activation of the inflammasome machinery. Signal 2 is delivered by a wide range of stimuli, which range from pathogen-derived molecules such as flagellin and cytosolic DNA, and non-pathogen-derived particulates such as uric acid crystals. The above two pathways appear to provide the minimum requirements for inflammasome activation; however, their activation is associated with an acute production of IL-1β, which is significantly resolved within 24 h [3] . Inflammasome activation is, however, also firmly established to have an important role in a number of chronic inflammatory and fibrotic diseases. Sustained production of IL-1β could theoretically occur within the framework of the above pathways by a greater number, concentration or duration of exposure to ligands that initiate signal 1 and 2 pathways. However, it is well known that persistent exposure to pathogen associated molecular patterns (PAMPs) results in the development of a tolerogenic state, and signal 2 pathways such as ATP induce cell death [4] , [5] , [6] , [7] . We speculated that there are additional regulatory signals, which are independent of the ligands that provide signals 1 and 2. The additional advantage of such signals is that they may provide distinct functional information. With this question in mind, we tested the role of adenosine in the regulation of inflammasome activation. Adenosine biology is well suited to regulate inflammasome activity because extracellular adenosine concentrations are elevated in response to tissue damage, and adenosine is rapidly removed from tissues by cellular uptake and adenosine deaminase-mediated metabolism [8] . This provides for a rapidly responsive mechanism that signals local tissue ischaemia and injury. Adenosine, however, has not been considered as a danger associated molecular patterns (DAMP) because it coordinates the adaptive responses to tissue injury in many ways in addition to inflammation and, more importantly, because most of the immunological effects have been to reduce cytokine production, with the notable exception of IL-1β [9] , [10] , [11] . In this study we demonstrate that adenosine acting via the A 2A receptor is a key regulator of inflammasome activity. Concentrations of adenosine found during tissue injury increase the maximal amplitude and duration of the inflammasome response. Inflammasome regulation by adenosine does not replace either signal 1 or 2 but regulates inflammasome activity initiated by a wide range of PAMPs and DAMPs. A cAMP/PKA (protein kinase A)/CREB (cAMP response element-binding protein)/HIF-1α (hypoxia-inducible factor-1α) signalling downstream of the A2A receptor is activated, and results in the upregulation of Pro-IL-1β and NLRP3, and greater caspase-1 activation. In addition to the regulation of inflammasome activity by pathological concentrations of adenosine, there is a requirement for physiological levels of adenosine for maximal IL-1β production. Finally, after macrophages have received signals 1 and 2, adenosine can regulate further IL-1β production, without the need for either initiating signal. This demonstrates that such cells are not simply tolerant or unresponsive to further signals but are in a post-activation state where they have switched from an initial DAMP-driven phenotype to a subsequent adenosine, cAMP-driven phenotype. Adenosine stimulates IL-1β in an inflammasome-dependent manner Initially we tested whether adenosine can increase IL-1β production above that produced by lipopolysaccharide (LPS) and ATP, both of which activate signals 1 and 2, respectively. The combination of LPS and ATP resulted in a high level of IL-1β production as assayed 5 h after ATP, and this was significantly increased by adenosine ( Fig. 1a ). To confirm that metabolites such as inosine produced via the degradation of adenosine were not responsible for the elevated IL-1β, the metabolism of adenosine from cellular sources was inhibited by using the adenosine deaminase inhibitor EHNA (erythro-9-(2-hydroxy-3-nonyl) adenine, and this also resulted in a significant increase in IL-1β production ( Fig. 1a ) [12] . Of note, adenosine and EHNA in the absence of either LPS or ATP did not result in any detectable IL-1β. To determine the effect of experimentally reducing adenosine concentration, adenosine deaminase was added, resulting in a significant reduction in IL-1β release ( Fig. 1a ). 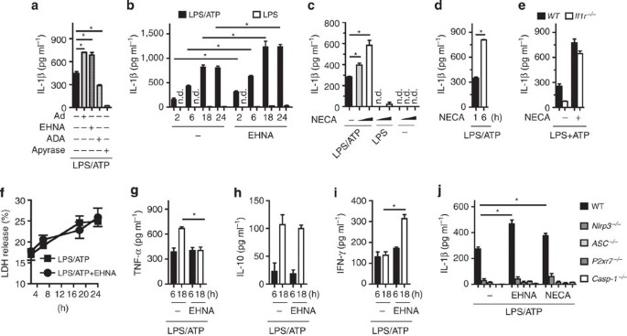Figure 1: Adenosine stimulates IL-1β production in an NLRP3 inflammasome-dependent manner. Murine PECs were obtained from wild-type (WT) mice (a–d,f–i),Il1r−/−(e) orNlrp3−/−,ASC−/−,P2xr7−/−orCaspase-1−/−mice (j) and were primed with LPS for 16 h. (a) This was followed by treatment for 1 h with adenosine (Ad, 100 μM), adenosine deaminase inhibitor (EHNA, 10 μM), adenosine deaminase (ADA, 10 U ml−1) or ATP diphosphohydrolase (Apyrase, 10 U ml−1), (b,f–i). Pan-adenosine agonist (NECA, 1 μM, 10 μM) (c,e) or (d) by NECA for 1 and 6 h and were then pulsed with ATP for 20 min. Enzyme-linked immunosorbent assay (ELISA) of IL-1β, TNF-α, IL-10 and IFN-γ secretion were measured in cell supernatants after pulsing with ATP for 5 h (a,c–e,j) or indicated time course. (b,g–i). Lactate dehydrogenase (LDH) assay was performed after pulsing with ATP as indicated time course (f). Data are expressed as the mean±s.d. from at least three independent experiments. *P<0.05 determined by Student’st-test. Figure 1: Adenosine stimulates IL-1β production in an NLRP3 inflammasome-dependent manner. Murine PECs were obtained from wild-type (WT) mice ( a – d , f – i ), Il1r −/− ( e ) or Nlrp3 −/− , ASC −/− , P2xr7 −/− or Caspase-1 −/− mice ( j ) and were primed with LPS for 16 h. ( a ) This was followed by treatment for 1 h with adenosine (Ad, 100 μM), adenosine deaminase inhibitor (EHNA, 10 μM), adenosine deaminase (ADA, 10 U ml −1 ) or ATP diphosphohydrolase (Apyrase, 10 U ml −1 ), ( b , f – i ). Pan-adenosine agonist (NECA, 1 μM, 10 μM) ( c , e ) or ( d ) by NECA for 1 and 6 h and were then pulsed with ATP for 20 min. Enzyme-linked immunosorbent assay (ELISA) of IL-1β, TNF-α, IL-10 and IFN-γ secretion were measured in cell supernatants after pulsing with ATP for 5 h ( a , c – e , j ) or indicated time course. ( b , g – i ). Lactate dehydrogenase (LDH) assay was performed after pulsing with ATP as indicated time course ( f ). Data are expressed as the mean±s.d. from at least three independent experiments. * P <0.05 determined by Student’s t -test. Full size image A time course was performed, and a sustained increase in IL-1β production by inhibition of adenosine deaminase was demonstrated ( Fig. 1b ). To further confirm that adenosine metabolites were not responsible for the increase in IL-1β via some other pathways, the non-degradable pan-adenosine receptor agonist NECA (5′-N-ethylcarboxamidoadenosine) was used, and also stimulated an increase in IL-1β production in LPS and ATP, and time-dependent manner ( Fig. 1c ). The IL-1 receptor uses the same Myd88 adaptor protein used by most TLRs and can increase IL-1β production via an autocrine loop [13] . To rule out that NECA was enhancing this autocrine pathway, we demonstrated that NECA can increase IL-1β production in macrophages from wild-type and IL-1 receptor-deficient mice to a similar degree ( Fig. 1e ) [13] . We next tested whether this phenomenon had applicability to other types of macrophages. LPS and ATP induced stimulation of bone marrow-derived macrophages and Kupffer cells (KCs), resulting in the production of IL-1β, and this was significantly increased by NECA ( Supplementary Fig. S1 ). Cell death was examined by the assay of lactate dehydrogenase release and did not show correlation with the secretion of IL-1β in the presence or absence of EHNA, indicating that differences in macrophage survival are not the reason for the increased IL-1β production ( Fig. 1f ). The effect of the adenosine pathway on the production of other cytokines was tested and the inhibition of adenosine deaminase resulted in a reduction in the production of tumour necrosis factor (TNF)-α, no effect on IL-10 and an increase in IFN-γ ( Fig. 1g–i ). We next tested whether the observed increase in IL-1β production was dependent on caspase-1, NLRP3, ASC and P2x7 receptor. In the absence of any of these molecules, stimulation of the adenosine signal by adding the pan-adenosine receptor agonist (NECA) or inhibiting adenosine deaminase (EHNA) did not result in significant production of IL-1β by LPS and ATP ( Fig. 1j ). NECA also increased IL-1β production by the combination of LPS and monosodium urate (MSU) crystals ( Supplementary Fig. S2a ). This was supported by data from different manipulations with the inhibition of adenosine metabolism resulting in an increase in CpG-B- and ATP-induced increase in IL-1β ( Supplementary Fig. S2b ). The reverse question of the contribution of A 2A receptor signalling to IL-1β production was tested by using the A 2A receptor antagonist ZM241385 in inflammasome activation by a variety of stimuli (CpG-B and ATP, Pam3 and ATP, LPS and beads, LPS and MSU and liver cell lysate) ( Supplementary Fig. S2c–g ). Finally, the contribution of A 2A receptor signalling in vivo was tested in the inflammasome-dependent model of MSU induced intraperitoneal sterile inflammation, which demonstrated a significant reduction in the presence of A 2A receptor antagonism ( Supplementary Fig. S2h ). These data show that activation of an adenosine pathway enhances the amount and duration of LPS and ATP induced IL-1β production in a NLRP3 inflammasome-dependent manner, and this is not because of an IL-1β autocrine loop. A 2A receptor activation amplifies signal 1 and 2 pathways There are four identified adenosine receptors (A 1 , A 2A , A 2B and A 3 ). These receptors are widely distributed and are coupled to stimulatory (A 2A and A 2B ) or inhibitory (A 1 and A 3 ) adenylate cyclases [9] , [11] . NECA increased IL-1β production, and this was inhibited by A 2A R antagonist (ZM241385), but not by A 1 R (DPCPX)-, A 2B R (MRS1706)- and A 3 R (MRS1523)-specific receptor antagonists ( Fig. 2a ). This result was replicated by examining the ability of an A 2A receptor agonist (CGS21680) to increase IL-1β production to a comparable degree to NECA and EHNA. All of these stimuli were inhibited by ZM241385 ( Fig. 2b ). Lactate dehydrogenase assay indicates that the inhibitory function of ZM241385 on LPS- and ATP-induced IL-1β secretion was not because of its cell toxicity ( Fig. 2c ). To confirm the role of the A 2A receptor, the ability of stimulation of the adenosine pathway to increase IL-1β production was tested in macrophages from A 2A receptor-deficient mice ( Adora2a −/− ). In the absence of A 2A receptor, there was virtually no production of IL-1β by LPS and ATP, and this was not increased by the stimulation of several components related to broad activation of adenosine pathways ( Fig. 2d ). To identify whether the increased production of IL-1β was because of adenosine-induced stimulation of signals 1 and 2, we initially examined upregulation of the Il1b gene in peritoneal macrophages from wild-type and A 2A -deficient mice in response to CGS21680 ( Fig. 2e ). The requirement for A 2A receptor was confirmed by a conventional strain of Adora2a knockout mice and Adora2a flox/flox /Lysozyme M-(LysM)-Cre ( A 2A R-cKO ) mice, which had significant reduction in A 2A receptor expression in the macrophages ( Supplementary Fig. S3 ); the macrophage from both strains had significantly less upregulation of the Il1b mRNA in response to LPS ( Fig. 2e ). To examine the role of A 2A receptor activation on signal 2-activated inflammasome pathway, we examined the effect of activation of A 2A receptor on the formation of active caspase-1. The A 2A receptor agonist CGS21680 alone did not result in detectable active caspase-1 ( Fig. 2g ). In response to LPS/ATP, active caspase-1 was detected, and this was decreased by blocking A 2A receptor with ZM241385 and increased by activating A 2A receptor with CGS21680. The increase in active caspase-1 by CGS21680 was also inhibited by ZM241385. In addition, the clear reduction in active caspase-1 was also detected in A 2A R-cKO macrophages in response to LPS/ATP ( Fig. 2h ). Collectively, these data show that adenosine-induced increase in LPS- and ATP-stimulated IL-1β production is via A 2A receptor and is because of an increase in both signal 1 and signal 2 pathways. 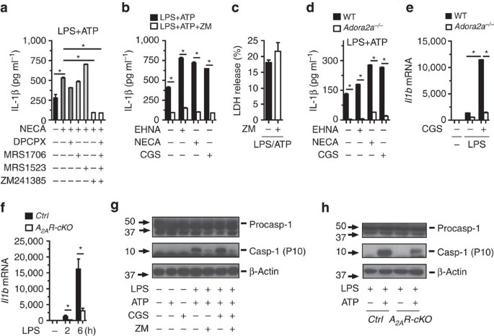Figure 2: Adenosine mediates increase in IL-1β via the A2Areceptor and amplifies signal 1 and signal 2 pathways. (a) LPS-primed PECs were treated with NECA (10 μM) in the presence or absence of three different adenosine receptor antagonists for A1(DPCPX, 10 nM), A2A(ZM241385, 10 μM), A2B(MRS1706, 10 nM), A3(MRS1523, 5 μM) or their combinations for 1 h and were pulsed with ATP for 20 min. (b) A2Areceptor-specific agonist (CGS21680) and antagonist ZM241385 increase and block IL-1β production, respectively. (c) LDH release in PECs showed no difference in the presence or absence of ZM241385 as sampled fromb. (d) PECs from A2Areceptor-deficient cells have low IL-1β production, which is not increased by NECA and CGS21680. (e) CGS21680 increases the induction ofIl1bmRNA expression, and this was decreased in A2Areceptor-deficient cells. (f) Loss of the A2Areceptor in macrophages results in much lower levels ofIl1bmRNA expression in response to LPS. (g) CGS21680 and ZM241385 increase and decrease production of cleaved caspase-1. (h) The production of cleaved caspase-1 is decreased in A2Areceptor-deficient macrophages. Data are expressed as the mean±s.d. from at least three independent experiments. Immunoblots shown are representative results from at least three independent experiments. *P<0.05 determined by Student’st-test. Figure 2: Adenosine mediates increase in IL-1β via the A 2A receptor and amplifies signal 1 and signal 2 pathways. ( a ) LPS-primed PECs were treated with NECA (10 μM) in the presence or absence of three different adenosine receptor antagonists for A 1 (DPCPX, 10 nM), A 2A (ZM241385, 10 μM), A 2B (MRS1706, 10 nM), A 3 (MRS1523, 5 μM) or their combinations for 1 h and were pulsed with ATP for 20 min. ( b ) A 2A receptor-specific agonist (CGS21680) and antagonist ZM241385 increase and block IL-1β production, respectively. ( c ) LDH release in PECs showed no difference in the presence or absence of ZM241385 as sampled from b . ( d ) PECs from A 2A receptor-deficient cells have low IL-1β production, which is not increased by NECA and CGS21680. ( e ) CGS21680 increases the induction of Il1b mRNA expression, and this was decreased in A 2A receptor-deficient cells. ( f ) Loss of the A 2A receptor in macrophages results in much lower levels of Il1b mRNA expression in response to LPS. ( g ) CGS21680 and ZM241385 increase and decrease production of cleaved caspase-1. ( h ) The production of cleaved caspase-1 is decreased in A 2A receptor-deficient macrophages. Data are expressed as the mean±s.d. from at least three independent experiments. Immunoblots shown are representative results from at least three independent experiments. * P <0.05 determined by Student’s t -test. Full size image Adenosine supersedes LPS tolerance via a CAMP-PKA pathway The demonstration that adenosine signalling can increase not just the amplitude but also the duration of IL-1β production directly has an impact on the well-characterized phenomenon of LPS tolerance [5] , [6] . In this phenomenon, exposure to LPS results in hypo-responsiveness to subsequent stimulation by LPS and other TLR agonists and occurs in-part by a lack of upregulation in pro-IL-1β [5] . We tested the ability of activation of the adenosine pathway to regulate Pro-IL-1β induction from peritoneal macrophages (PECs) with previous exposure to LPS. As expected, 3 h after initial stimulation of PECs with LPS (Stim) there is upregulation of the Il1b mRNA expression ( Fig. 3a ). PECs pretreated with LPS (Pri) for 16 h had low levels of pro-IL-1β and did not respond to a repeat stimulation with LPS ( Fig. 3a ). In sharp contrast to a lack of response of LPS-pretreated PECs to repeat LPS stimulation, there was a dramatic increase in Il1b mRNA expression in response to either NECA or CGS21680 ( Fig. 3a ). These results demonstrate that after an initial signal 1, when PECs are unresponsive to further signal 1 ligands, they become highly responsive to adenosine by upregulating Il1b . We next tested whether this ability of adenosine to supersede LPS tolerance was true for other cytokines. Over 6- and 24-h CGS21680 and NECA were able to increase the expression levels of Il-1b, ll-6 , Il-4 but not tnfa ( Supplementary Fig. S4a–d ). As sustained, inflammasome activation has also been shown to be important in chronic tissue fibrosis and remodelling we examined the expression of relevant genes and found a consistent ability of CGS21680 and NECA to supersede LPS tolerance for tissue inhibitor of metalloproteinases-1, vascular endothelial growth factor and Glucose transporter 1 ( Supplementary Fig. S4e–h ). This is consistent with previous data showing that adenosine increases tissue inhibitor of metalloproteinases-1 in IL-4- or IL-13-activated macrophages [14] . In contrast, other antimicrobial gene such as macrophage receptor Marco was upregulated by adenosine signal activation, and this was found to be dependent on A 2A and IL-1 receptor signalling ( Supplementary Fig. S5a–f ). 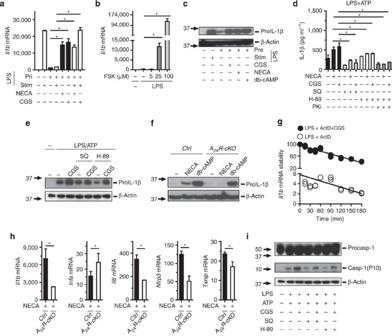Figure 3: Adenosine supersedes LPS-induced tolerance and increases IL-1β production by upregulating transcription of pro-IL-1β via the CAMP-PKA pathway. PECs were used in all of the following experiments. (a) Primed (pri) with LPS (100 ng ml−1) for 16 h followed by stimulation (stim) with LPS (100 ng ml−1), or NECA (10 μM) or CGS21680 (10 μM) in the presence or absence of LPS (100 ng ml−1) for 6 h. (b) Treated with forskolin for 6 h as indicated doses with and without LPS priming. (c) Treated with or without NECA (10 μM), CGS21680 (10 μM) or db-cAMP (200 μM) for 6 h. (d) LPS primed and treated with NECA or CGS21680 in the presence and absence of SQ22536, H-89 and PKi. (e) Primed with LPS for 16 h and treated with ATP for 20 min, followed by CGS21680 in the presence or absence of the adenylyl cyclase and PKA inhibitors SQ22536 and H-89. (f) Primed with LPS and treated with or without NECA (10 μM) or db-cAMP (200 μM) for 6 h. (g) Treated with or without CGS21680 (10 μM) for 3 h, and transcription was stopped by adding 5 μg ml−1actinomycin D, and RNA samples collected at indicated time points. (h) LPS-primed PECs obtained from wild-type orA2AR-cKOmice were stimulated with NECA (10 μM) for 6 h. The cells were harvested and RNA was isolated after each treatment and the gene expression ofIl1band other genes as indicated quantified using real-time PCR using specific primers. (i) Primed with LPS for 16 h and treated with ATP for 20 min, followed by CGS21680 in the presence or absence of SQ22536 or H-89. Immunoblot analysis of the pro-IL-1β caspase-1 in cell lysate was performed by specific anti-IL-1β and anti-caspase-1 p10 antibodies (c,e,f,i). Data are expressed as the mean±s.d. from three independent experiments. Immunoblots shown are representative results from at least three independent experiments. *P<0.05 determined by Student’st-test. Figure 3: Adenosine supersedes LPS-induced tolerance and increases IL-1β production by upregulating transcription of pro-IL-1β via the CAMP-PKA pathway. PECs were used in all of the following experiments. ( a ) Primed (pri) with LPS (100 ng ml −1 ) for 16 h followed by stimulation (stim) with LPS (100 ng ml −1 ), or NECA (10 μM) or CGS21680 (10 μM) in the presence or absence of LPS (100 ng ml −1 ) for 6 h. ( b ) Treated with forskolin for 6 h as indicated doses with and without LPS priming. ( c ) Treated with or without NECA (10 μM), CGS21680 (10 μM) or db-cAMP (200 μM) for 6 h. ( d ) LPS primed and treated with NECA or CGS21680 in the presence and absence of SQ22536, H-89 and PKi. ( e ) Primed with LPS for 16 h and treated with ATP for 20 min, followed by CGS21680 in the presence or absence of the adenylyl cyclase and PKA inhibitors SQ22536 and H-89. ( f ) Primed with LPS and treated with or without NECA (10 μM) or db-cAMP (200 μM) for 6 h. ( g ) Treated with or without CGS21680 (10 μM) for 3 h, and transcription was stopped by adding 5 μg ml −1 actinomycin D, and RNA samples collected at indicated time points. ( h ) LPS-primed PECs obtained from wild-type or A 2A R-cKO mice were stimulated with NECA (10 μM) for 6 h. The cells were harvested and RNA was isolated after each treatment and the gene expression of Il1b and other genes as indicated quantified using real-time PCR using specific primers. ( i ) Primed with LPS for 16 h and treated with ATP for 20 min, followed by CGS21680 in the presence or absence of SQ22536 or H-89. Immunoblot analysis of the pro-IL-1β caspase-1 in cell lysate was performed by specific anti-IL-1β and anti-caspase-1 p10 antibodies ( c , e , f , i ). Data are expressed as the mean±s.d. from three independent experiments. Immunoblots shown are representative results from at least three independent experiments. * P <0.05 determined by Student’s t -test. Full size image The A 2A receptor is coupled to a stimulatory adenylate cyclase, which results in the upregulation of cAMP and activation of protein kinase A [8] . To test this pathway, we used the adenylate cyclase activator forskolin, which induced the induction of the Il1b gene in a dose-dependent manner ( Fig. 3b ). This was confirmed by directly using a stable analogue of cAMP (N 6 ,2′-O-Dibutyryladenosine 3′,5′-cyclic monophosphate sodium salt (db-cAMP)), which along with NECA and CGS21680 induced the upregulation of Pro-IL-1β ( Fig. 3c ). To test the requirement for the adenylate cyclase/cAMP/PKA pathway on A 2A receptor signal-induced IL-1β production, an adenylate cyclase inhibitor (SQ22536) was tested and was able to block the increase in IL-1β induced by CGS21680 and EHNA ( Fig. 3d ) [15] . We next tested the requirement of PKA downstream of cAMP activation using the specific inhibitors of H-89 and PKI 14-22 amide (PKi). PKA inhibition significantly reduced the IL-1β production in response to NECA and CGS21680 ( Fig. 3d ). This was confirmed for the pro-IL-1β protein level using western blot ( Fig. 3e ). We next confirmed that the lack of response in cells from A 2A receptor-deficient mice ( Fig. 2e ) was not because of developmental effects by testing the ability of db-cAMP to increase pro-IL-1β protein levels in A 2A R-cKO mice ( Fig. 3f ). To determine whether the greater amounts of Pro-IL-1β transcripts after A 2A receptor activation were because of increased transcript stability, we used actinomycin D to inhibit transcription and examined the effect of CGS21680 on the loss of Pro-IL-1β transcript. The rate of loss of Il1b mRNA expression was identical, showing that CGS21680 did not affect transcript stability ( Fig. 3g ). To confirm the role of A 2A receptor in increasing TLR-induced Pro-IL-1β upregulation, the response of macrophages from A 2A receptor-deficient mice was tested. In the absence of A 2A receptor, there was minimal increase in LPS-induced upregulation of Il1b mRNA expression ( Fig. 3h ). Finally, we tested the role of adenosine signalling and A 2A receptor in the changes associated with a number of cytokine- and inflammasome-related transcripts ( Fig. 3h ). In contrast to decreased Il1b and Il6 mRNA in A 2A receptor-deficient cells, there was a higher level of tnfa . Of interest, there were also lower levels of Nlrp3 and Txnip transcripts in A 2A receptor-deficient cells. This prompted us to test whether the adenylate cyclase/cAMP/PKA pathway was also required for the A 2A receptor-induced increase in active caspase-1. This was the case, with the CGS21680-induced upregulation in LPS/ATP-induced active caspase-1 being reduced by SQ22536 and H-89 ( Fig. 3i ). Interestingly, in contrast to these findings, under non-LPS tolerogenic condition, adenosine-cAMP signalling did not show increase in IL-1β secretion by inflammasome activation, indicating distinct role of adenosine in deriving IL-1β production ( Supplementary Fig. S6a–d ). Collectively, these data show that adenosine signalling can supersede LPS tolerance of signal 1 via the A 2A receptor and does so via an adenylate cyclase/cAMP/PKA-mediated pathway. Adenosine induces pro-IL-1β via CREB and HIF-1α To understand the link between PKA activation and Pro-IL-1β upregulation, we and others identified HIF-1α response elements in the human and mouse Il1b promoter ( Fig. 4a ) [16] . This led us to consider that HIF-1α activation may be a central step in upregulating Pro-IL-1β. We assayed whether A 2A receptor activation resulted in upregulation of the Hif1a mRNA, and found this to be the case ( Fig. 4b ). The HIF-1α inhibitor CAY10585 was able to significantly decrease adenosine agonist-induced Il1b expression and IL-1β production ( Supplementary Fig. S7a,b ). To specifically test the role of HIF-1α in A 2A receptor activation-induced upregulation of Il1b mRNA, HIF-1 α flox/flox /Lysozyme M (LysM)-Cre mice ( HIF-1 α -cKO ) were generated, and high deletion efficiency was demonstrated in bone marrow-derived macrophages ( Supplementary Fig. S3b ). LPS-primed HIF-1 α -cKO macrophages had significantly less A 2A receptor stimulation-induced upregulation of Il1b than wild-type macrophages ( Fig. 4c ). We further demonstrated that LPS-primed HIF-1 α -cKO macrophages had significantly less A 2A receptor stimulation-induced upregulation of Nlrp3 and Txnip mRNAs than wild-type macrophages ( Supplementary Fig. S7c,d ). 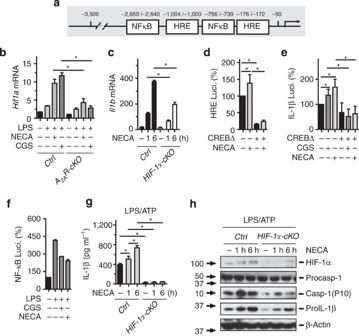Figure 4: Adenosine mediates increase in pro-IL-1β via a HIF-1α-dependent pathway. (a) Consensus NF-κB and HRE-binding sites in the IL-1β promoter. (b) LPS-primed PECs obtained fromA2AR-cKOand controls were stimulated with or without NECA or CGS21680. (c) LPS-primed PECs obtained fromHIF-1α-cKOand controls were stimulated with or without NECA at time points as indicated. Cells were harvested and RNA isolated after each treatment and gene expression ofIl1bandHif-1α quantified using real-time PCR. (d) THP-1 cells were transfected with HRE-promoter luciferase construct and β-galactosidase plasmid in the presence or absence of CREB-dominant-negative plasmid (CREBΔ), and then primed with LPS/PMA followed by NECA. (e) THP-1 cells were transfected with human IL-1β promoter luciferase construct and β-galactosidase plasmid in the presence or absence of CREBΔ, and then primed with LPS/PMA followed by CGS21680 or NECA. Luciferase activities were measured and normalized to β-galactosidase activity and normalized with controls. Data are mean±s.d. of triplicate cultures and are representative of three independent experiments. (f) CD14-MD2-TLR4-HEK 293 cells were transfected with NF-κB promoter luciferase construct and Renilla luciferase (Rluc) control reporter vector, and then treated with CGS21680, NECA or ZM241385 in the presence of LPS. Luciferase activities were measured and normalized to Rluc activity and the normalized value with controls as indicated. Data are mean±s.d. of triplicate cultures and are representative of three independent experiments forb–f. (g) LPS-primed PECs obtained fromHIF-1α-cKOand controls were treated with or without NECA at different time points as indicated followed by pulsing with ATP. Cell supernatants were collected in 5 h after ATP-pulsing. IL-1β was measured in cell supernatant using ELISA. Data are expressed as the mean±s.d. from three independent experiments. (h) LPS-primed PECs obtained fromHIF-1α-cKOand control mice were treated with or without NECA at different time points as indicated, followed by pulsing with ATP. Cell lysates were collected after ATP-pulsing. HIF-1α, pro-caspase-1, Caspase-1 and pro-IL-1β were measured by western blot. Immunoblots shown are representative results from at least three independent experiments. *P<0.05 determined by Student'st-test. Figure 4: Adenosine mediates increase in pro-IL-1β via a HIF-1α-dependent pathway. ( a ) Consensus NF-κB and HRE-binding sites in the IL-1β promoter. ( b ) LPS-primed PECs obtained from A 2A R-cKO and controls were stimulated with or without NECA or CGS21680. ( c ) LPS-primed PECs obtained from HIF-1 α -cKO and controls were stimulated with or without NECA at time points as indicated. Cells were harvested and RNA isolated after each treatment and gene expression of Il1b and Hif-1 α quantified using real-time PCR. ( d ) THP-1 cells were transfected with HRE-promoter luciferase construct and β-galactosidase plasmid in the presence or absence of CREB-dominant-negative plasmid (CREBΔ), and then primed with LPS/PMA followed by NECA. ( e ) THP-1 cells were transfected with human IL-1β promoter luciferase construct and β-galactosidase plasmid in the presence or absence of CREBΔ, and then primed with LPS/PMA followed by CGS21680 or NECA. Luciferase activities were measured and normalized to β-galactosidase activity and normalized with controls. Data are mean±s.d. of triplicate cultures and are representative of three independent experiments. ( f ) CD14-MD2-TLR4-HEK 293 cells were transfected with NF-κB promoter luciferase construct and Renilla luciferase (Rluc) control reporter vector, and then treated with CGS21680, NECA or ZM241385 in the presence of LPS. Luciferase activities were measured and normalized to Rluc activity and the normalized value with controls as indicated. Data are mean±s.d. of triplicate cultures and are representative of three independent experiments for b – f . ( g ) LPS-primed PECs obtained from HIF-1 α -cKO and controls were treated with or without NECA at different time points as indicated followed by pulsing with ATP. Cell supernatants were collected in 5 h after ATP-pulsing. IL-1β was measured in cell supernatant using ELISA. Data are expressed as the mean±s.d. from three independent experiments. ( h ) LPS-primed PECs obtained from HIF-1 α -cKO and control mice were treated with or without NECA at different time points as indicated, followed by pulsing with ATP. Cell lysates were collected after ATP-pulsing. HIF-1α, pro-caspase-1, Caspase-1 and pro-IL-1β were measured by western blot. Immunoblots shown are representative results from at least three independent experiments. * P <0.05 determined by Student's t -test. Full size image A direct link between PKA activation and HIF-1α upregulation is provided by CREB, which enhances two C-terminus transactivating domains in HIF-1α [17] . The requirement for CREB in adenosine-induced upregulation of HIF-1α was tested by the transfection of THP-1 human monocyte cell line with the HRE-promoter luciferase construct and β-galactosidase plasmid in the presence or absence of CREB-dominant-negative plasmid (CREBΔ) for 24 h and then primed with LPS/PMA for 16 h followed by NECA treatment over 8 h. As predicted, an adenosine stimulus resulted in HRE reporter luciferase activity, and this was inhibited by the presence of the dominant-negative CREB plasmid ( Fig. 4d ) [18] , [19] . In an analogous manner, transfection of the IL-1β promoter luciferase construct and β-galactosidase plasmid in the presence or absence of CREB-dominant-negative form demonstrated a requirement for CREB signalling for the production of IL-1β ( Fig. 4e ) [20] . Transcriptional upregulation of Pro-IL-1β on initial LPS stimulation is via activation of the NF-κB pathway. We tested whether the subsequent transcriptional upregulation of Pro-IL-1β also uses this pathway and found that adenosine agonists do not increase activity of the NF-κB pathway above that already induced by LPS ( Fig. 4f ). This is in agreement with previous studies [21] , [22] . We finally confirmed that in the absence of HIF-1α there was a significant reduction at the protein level in pro-caspase-1, activated caspase-1, pro-IL-1β and ultimately active IL-1β ( Fig. 4g ). These data show that adenosine-induced upregulation of IL-1β is dependent on a CREB/HIF-1α pathway, which is distinct from the NF-κB pathway used for initial production of IL-1β in response to LPS. Liver injury is dependent on A 2A receptor in macrophages The above data show a requirement for adenosine signalling via the A 2A receptor for maximal production of IL-1β by macrophages in vitro . With tissue inflammation and injury, extracellular adenosine levels are known to increase by a variety of means from the basal levels below 1 μM to levels up to 100 mM [23] , [24] . We tested whether A 2A receptor-driven inflammasome activity was relevant in vivo and used two models of liver injury, one acute LPS-driven model where liver injury was assessed in 6 h after LPS, and a second model of sterile injury by a toxic metabolic insult to the liver by thioacetamide (TAA) in which injury was examined at days 1, 2 and 7. We used A 2A R-cKO mice that specifically delete the Adora2a gene in macrophages as described above. Liver immune populations were intact in these mice ( Supplementary Fig. S8 ). Six hours after LPS and D-galactosamine induced liver injury, there was significantly less haemorrhage and necrosis in the livers from A 2A R-cKO mice and this was confirmed by lower serum ALT values ( Fig. 5a ). Reduced activation of the inflammasome was confirmed by demonstrating that the whole liver had lower levels of Il1b mRNA, less active caspase-1, and that there were lower levels of serum IL-1β ( Fig. 5b–d ). To test the effect of increasing adenosine signalling in vivo , wild-type mice were treated with LPS in the presence or absence of the adenosine agonist NECA. The presence of NECA resulted in a significant elevation in serum ALT, whole-liver transcripts of Il1b , Il6 , Hif1a and Nlrp3 , and a reduction in the transcript for tnfa ( Supplementary Fig. S9 ). 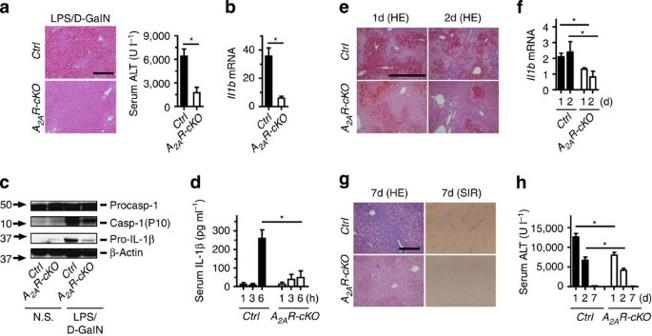Figure 5: Liver injury and fibrosis are dependent on A2Areceptor signalling in macrophages. (a)A2AR-cKOand control mice were injected intraperitoneally with LPS (1 mg kg−1) and D-galactosamine (500 mg kg−1) for 6 h followed by liver tissue and serum collection for H&E staining and ALT assay. (b) Liver RNA samples were collected and theIl1bgene assayed using real-time PCR using specific primers. (c) Liver tissue lysates were assayed for pro-caspase-1, cleaved caspase-1 (p10) and β-actin protein level using immunoblot analysis using specific antibodies. Data are expressed as the mean±s.d. from 10 to 11 mice from each group fora–d. (d) Serum was collected for measurement of IL-1β. (e)A2AR-cKOand control mice were injected intraperitoneally with single dose of TAA followed by liver tissue collection as indicated for H&E staining. (f) Liver RNA samples were collected and theIl1bgene was assayed using real-time PCR. (g) Liver tissue was also obtained on day 7 after TAA injection and stained with H&E and Sirius red for fibrosis. (h) Sera were collected and the serum ALT assay was performed (data are expressed as the mean±s.d. from five mice in each group). *P<0.05 determined by Student’st-test. Scale bars correspond to 500 μm. Figure 5: Liver injury and fibrosis are dependent on A 2A receptor signalling in macrophages. ( a ) A 2A R-cKO and control mice were injected intraperitoneally with LPS (1 mg kg −1 ) and D-galactosamine (500 mg kg −1 ) for 6 h followed by liver tissue and serum collection for H&E staining and ALT assay. ( b ) Liver RNA samples were collected and the Il1b gene assayed using real-time PCR using specific primers. ( c ) Liver tissue lysates were assayed for pro-caspase-1, cleaved caspase-1 (p10) and β-actin protein level using immunoblot analysis using specific antibodies. Data are expressed as the mean±s.d. from 10 to 11 mice from each group for a – d . ( d ) Serum was collected for measurement of IL-1β. ( e ) A 2A R-cKO and control mice were injected intraperitoneally with single dose of TAA followed by liver tissue collection as indicated for H&E staining. ( f ) Liver RNA samples were collected and the Il1b gene was assayed using real-time PCR. ( g ) Liver tissue was also obtained on day 7 after TAA injection and stained with H&E and Sirius red for fibrosis. ( h ) Sera were collected and the serum ALT assay was performed (data are expressed as the mean±s.d. from five mice in each group). * P <0.05 determined by Student’s t -test. Scale bars correspond to 500 μm. Full size image Toxic injury by TAA demonstrated maximal haemorrhage and necrosis on day 1. There was less liver haemorrhage and necrosis, and lower levels of liver Il1b mRNA and serum ALT in A 2A R-cKO mice ( Fig. 5e–h ). In addition to inflammation, inflammasome activity has been shown to be required for the development of the fibrotic response in many organs [25] , [26] , [27] . To assess whether fibrosis was also affected in the absence of A 2A receptor on tissue macrophages, liver tissues from 7 days after TAA were stained for collagen by Sirius Red. There was significantly less fibrosis in livers from A 2A R-cKO mice compared with the wild type ( Fig. 5g ). A sustained IL-1β production was also seen in liver tissue and serum after a course of repeated TAA injection in wild-type control but not A 2A R-cKO mice ( Supplementary Fig. S10a–c ). To further test the effect of increased adenosine signalling on fibrosis, wild-type and caspase-1-deficient mice were injected with TAA with and without co-injection of the adenosine agonist CGS21680. After 1 week, liver tissues were stained for collagen with Sirius Red. CGS21680 increased TAA-induced liver fibrosis and Timp1 expression in wild-type but not in caspase-1-deficient mice ( Supplementary Fig. S11a,b ). Collectively, these data confirm that adenosine-induced signalling via the A 2A receptor is important for in vivo activation of the inflammasome in acute and chronic injury. Original blots for the data shown are in Supplementary Fig. S12 . The current model of inflammasome activation in macrophages explains the initial steps in acute inflammation but is inadequate to explain how activity is sustained in chronic inflammation, repair and fibrosis [1] , [2] . The issue is not only the self-limited inflammatory response induced by signals 1 and 2 but also the unresponsiveness of macrophages to similar subsequent signals [5] , [6] . As macrophages are unresponsive to repeat exposure to the initiating signals, we reasoned that further signals are qualitatively different, with signals from tissue injury being attractive candidates. Adenosine is well known to regulate tissue responses to stress and injury via activation of four widely distributed receptors [9] , [11] . Adenosine levels rapidly increase in the extracellular environment in response to cell stress and death by release from cytosolic stores and sequential dephosporylation from ATP and are rapidly reduced by uptake and metabolism [11] , [23] , [24] . Manipulations that increase adenosine signalling result in increased release of IL-1β from conventionally activated PEC, and this is not because of enhancement of an IL-1-mediated positive feedback loop ( Fig. 1a–e ). Adenosine has a role concurrent with or after conventional inflammasome activation. The in vivo implications are that during and after inflammasome activation the ambient adenosine concentration regulates the duration of inflammasome activation and can restimulate it. Our data are consistent with the original in vivo data from A 2A receptor-deficient mice showing a lack of rise in serum IL-1β in response to LPS [10] . The contribution of A 2A receptor activation is to upregulate the transcript levels of Pro-IL-1β, NLRP3 and others. This means that an adenosine stimulus can upregulate both arms of signal 1 and 2 pathways, as demonstrated by greater levels of the pro-IL-1β protein and active caspase-1 ( Fig. 3e ). Furthermore, this is a broad response with adenosine increasing inflammasome activation in response to a range of TLR stimuli for signal 1, as well as ATP, monosodium urate and synthetic bead-induced activation of signal 2 ( Supplementary Fig. S2 ). Initial activation of PEC by LPS results in high levels of Pro-IL-1β, and subsequent exposure to LPS cannot stimulate a repeated elevation, which is the well-characterized phenomenon of LPS tolerance [5] , [6] . We now show that after initial activation, PEC will upregulate Pro-IL-1β and produce IL-1β in response to adenosine signals without further exposure to conventional signals 1 and 2. These PEC are clearly not unresponsive in a global way; rather after initial activation by LPS and ATP they have switched their phenotypes into a state in which Pro-IL-1β production is regulated by adenosine signals ( Fig. 3a ). This is better characterized as a post activation, rather than an unresponsive state. The effect of adenosine is however not uniform for all cytokines. In particular, adenosine results in downregulation of TNF-α production and does not alter the genes for most antimicrobial proteins ( Supplementary Fig. S5 ). The initial steps downstream of the A 2A receptor that are required for the increased IL-1β production are the signalling molecules cAMP and PKA ( Fig. 3b–f ) [28] . Detailed investigation [29] using HIF-1α inhibitors, reporter constructs and macrophage-specific knockouts demonstrates that the ability of adenosine signals to upregulate pro-IL-1β is dependent on HIF-1α and CREB, with CREB being proximal to HIF-1α ( Fig. 4b–d ). This is distinct from the NF-κB pathway utilized for pro-cytokine upregulation after initial TLR activation, which has previously been shown not to be reduced by adenosine signalling [21] , [22] , [30] . The prediction from these in vitro data is that in the absence of A 2A receptor signalling on macrophages, there will be reduced inflammasome activation, with less tissue injury and fibrosis. This was the case in an acute and sustained model of LPS- and TAA-induced liver injury ( Fig. 5 ). This provides valuable confirmation of the scale of the adenosine signal in vivo . In a number of experimental models, total A 2A receptor-deficient animals have greater organ injury [31] , [32] . This apparent contradiction can be resolved if adenosine is simultaneously functioning to enhance macrophage-based inflammatory responses and providing parenchymal cell protection, with both being part of an integrated response to tissue injury by pathogens and sterile insults. In summary, we demonstrate that macrophages after receiving conventional signals 1 and 2 are dependent on adenosine via the A 2A receptor for initial and sustained inflammasome activity and IL-1β production. Conceptually, this is significant as it changes our interpretation of a lack of cytokine response by macrophages after LPS exposure from the cell being in an unresponsive state, to it being in a post-activation state, which is regulated by a different set of signals. Mechanistically and therapeutically, this is significant as it requires a clearer understanding if tissue injury is because of the initial inflammasome activation, or is because of maintenance of the activation state. Different antagonist and inhibitors will be effective to limit each of these. Animals and macrophages C57BL/6 mice were purchased from the National Cancer Institute. ASC −/− , Caspase-1 −/− , Nlrp3 −/− and P2xr7 −/− mice have been described previously (1). A2ora2a flox/flox and LysM cre mice were purchased from Jackson Laboratories. HIF1a flox/flox mice were kindly provided by Dr Ruslan M. Medzhitov (Yale University). Adora2a −/− mice were maintained at the animal facility of New York School of medicine according to the regulations of Animal Care and Use Committee of the New York University. All procedures were performed in accordance with the regulations adopted by the National Institutes of Health and approved by the Animal Care and Use Committee of the Yale University. Seven- to 12-week-old male mice with a variety of genetic manipulations were used in most experiments. The number of mice in each experimental group was chosen based on previous experience with these experimental models. Mouse PECs were isolated by peritoneal lavage 3 days after intraperitoneal injection of 4% thioglycollate solution (B2551, Fluka). Cells were plated at the density of 3 × 10 6 cells in 12-well dishes and non-adherent cells were removed after 3 h. Cells primed overnight with 100 ng ml −1 LPS or 10 ng ml −1 Pam3CSK4 were treated with various chemicals, followed by stimulation. Cells were cultured in Dulbecco’s modified Eagle’s medium medium complemented with 10% fetal bovine serum, penicillin/streptomycin and L -glutamine. Mouse bone marrow-derived macrophages were isolated from bone marrow cells and were differentiated for 7 days in complete RPMI-1640 medium supplemented with 2 mM L -glutamine, 100 U ml −1 penicillin, 100 μg ml −1 streptomycin, 50 μM 2-mercaptoethanol (all from Invitrogen), 10% heat-inactivated fetal bovine serum and 20 ng ml −1 M-CSF (PeproTech). KCs were isolated by the density gradient separation of Optiprep (Sigma), and then plates were gently washed and media was replenished after seeding cells for 2 h to raise KC purity. Reagents ATP, LPS from Salmonella minnesota Re-595, Forskolin (cAMP analogue), SQ22536 (AC inhibitor), H-89 (PKA inhibitor), MRS1523 (A 3 antagonist), adenosine, EHNA (adenosine deaminase inhibitor), NECA (nonselective adenosine receptor agonist), db-cAMP and Apyrase were obtained from Sigma (St. Louis, MO, USA). Adenosine deaminase was obtained from Worthington Biochemical corporation (Lakewood, NJ, USA). CGS21680 (A 2A agonist), DPCPX (A 1 antagonist), ZM241385 (A 2A antagonist) and MRS1706 (A 2B antagonist) were obtained from TOCRIS (Ellisville, MI, USA). Nigericin was purchased from Calbiochem, Pam3CSK4 and type B CpG oligonucleotide (ODN 1668, CpG-B) were purchased from Invivogen (San Diego, CA, USA). CAY10585 (HIF-1α inhibitor) was purchased from Cayman Chemical (Ann Arbor, MI, USA). TRIZOL and Dulbecco’s modified Eagle’s medium were purchased from GIBCO/Invitrogen (Carlsbad, CA, USA). All reagents were of the highest quality grade commercially available. MSU crystals were produced as previously described (2). Briefly, 4 mg ml −1 uric acid (Sigma-Aldrich) was dissolved in 0.1 M borate buffer by continuously adjusting the pH to 8.0. The solution was filtered, and the crystals precipitated after 7 days were washed twice with absolute alcohol and once with acetone and air-dried in a tissue culture hood before use. Quantitative real-time RT–PCR Total RNA was extracted using TRIZOL reagent (Invitrogen), and cDNA was generated with an oligo (dT) primer and the Superscript II system (Invitrogen) followed by analysis using LightCycler 480 system (Roche, Indianapolis, IN, USA). q-PCR was performed for Il1b using commercial primer–probe sets (Applied Biosystems Inc.) with DNA master Mix (Roche). Expression of GAPDH was used to standardize the samples, and the results were expressed as a ratio relative to control; q-PCR was performed for tnfa , Il6, Txnip, Nlrp3, Hif1a, Timp1 , using LightCycler 480 SYBR Green I master mix (Roche). Results were normalized based on the expression of β-actin. Primer sequences are listed in Supplementary Table S1 . Transfection and luciferase reporter assay THP-1 cells (Sigma-Aldrich) were transiently transfected with human IL-1β promoter (−1 to −4,000) luciferase or HRE-luciferase construct in the presence of CREBΔ plasmid or empty vector. For each transfection, the total of 2.0 μg of plasmid was mixed with 200 μl of Opti-MEM I medium (without serum and antibiotics) and 8.0 μl of X-tremeGENE HP DNA Transfection Reagent (Roche) according to the manufacturer’s instructions. The mixture was incubated at room temperature for 20 min and added to six-well plates containing cells and complete medium in a dropwise manner. The cells were incubated for 48 h and harvested using reporter lysis buffer (Promega) for determination of luciferase activity. Cells were co-transfected with β-galactosidase reporter plasmid to normalize experiments for transfection efficiency. 293T cells (InvivoGen) were transiently transfected with NF-κB promoter luciferase reporter construct together with Renilla luciferase (Rluc) control reporter vector by Lipofectamine 2000 reagent. All the luciferase activities were measured and normalized to Rluc or β-galactosidase activity, and the normalized value with the percentage of control group was indicated. Flow cytometry Liver non-parenchymal cells were isolated and antibodies were conjugated to FITC, PE, allophycocyanin specific for CD11b (1:200, M1/70), GR-1 (1:200, RB6-8C5) (BD Biosciences—Pharmingen), Ly6-C (1:200, HK1.4) and F4/80 (1:200, BM8, eBioscience). Stained cells were analysed using FACScalibur (BD Biosciences). Cytokine enzyme-linked immunosorbent assay measurements Primed macrophages were both pulsed for 20 min with 5 mM ATP or 10 μM nigericin and left untreated until culture supernatants were collected. Secretion of IL-1β was determined using enzyme-linked immunosorbent assay (R&D Systems). Western blot analysis Liver tissue lysates or macrophages were lysed in RIPA buffer (10 mM phosphate buffer pH 7.4, 150 mM NaCl, 1% NP-40, 0.5% sodium deoxycholate, 0.1% SDS) supplemented with complete protease inhibitor cocktail (Roche) and 2 mM dithiothreitol. Lysates were resolved in 4–12% Tris-glycine gradient gels (Invitrogen) and transferred to nitrocellulose (Invitrogen) by electroblotting. The following antibodies were used: rabbit anti-caspase-1 p10 (SC-514, Santa Cruz Biotechnology), goat anti-mouse IL-1β (BAF401, R&D Systems), Rabbit anti-mouse HIF-1α (NB100-449, Novus Biologicals, Littleton, CO, USA). Statistical analysis All data were expressed as mean±s.d. Student’s t -test was used for statistical evaluation of the results. Significance was set at P <0.05. How to cite this article: Ouyang, X. et al. Adenosine is required for sustained inflammasome activation via the A 2A receptor and the HIF-1α pathway. Nat. Commun. 4:2909 doi: 10.1038/ncomms3909 (2013).